An autonomous DNA nanomachine maps spatiotemporal pH changes in a multicellular living organism Structural DNA nanotechnology seeks to build synthetic molecular machinery from DNA. DNA nanomachines are artificially designed assemblies that switch between defined conformations in response to an external cue. Though it has proved possible to create DNA machines and rudimentary walkers, the function of such autonomous DNA-based molecular devices has not yet been achieved inside living organisms. Here we demonstrate the operation of a pH-triggered DNA nanomachine inside the nematode Caenorhabditis elegans . The nanomachine uses fluorescence resonance energy transfer to effectively map spatiotemporal pH changes associated with endocytosis in wild type as well as mutant worms, demonstrating autonomous function within the organismal milieu in a variety of genetic backgrounds. From this first demonstration of the independent functionality of a DNA nanomachine in vivo , we observe that rationally designed DNA-based molecular devices retain their in vitro functionality with quantitative precision. This positions DNA nanodevices as exciting and powerful tools to interrogate complex biological phenomena. A living cell is a combination of a large number of molecular devices working autonomously within the molecularly crowded cellular milieu in an orchestrated fashion to sustain and preserve life. A large number of these molecular devices are based on nucleic acid scaffolds, for example, riboswitches [1] , ribozymes [2] , transposons [3] , ribosomes [4] , cis -regulatory elements on DNA [5] , spliceosomes [6] , to name a few. Owing to the specificity and predictability of Watson-Crick base pairing, engineerability and the ability to form a rich repertoire of unusual structures based on their sequence and external triggers, nucleic acids have proven to be a remarkably powerful scaffold to build a variety of programmable synthetic nanomachines [7] . Examples include DNA tweezers, walkers and DNA-hybridization powered molecular motors [8] , [9] . Despite the existence of several highly effective, naturally occurring nucleic acid-based devices in vivo and an array of complex, synthetic DNA-based molecular devices in vitro , the functional application of such rationally designed artificial DNA-based nanodevices within a living organism is yet to be achieved. Previous work from our laboratory has outlined the construction and working of an autonomous DNA nanomachine that undergoes a conformational switch in response to pH changes [10] . This DNA nanomachine, called the I-switch, consists of two DNA duplexes connected to each other by a flexible hinge and bearing cytosine-rich single-stranded overhangs at the duplex termini ( Fig. 1a ). Upon protonation, these cytosine-rich overhangs unite with each other to form an I-motif [11] , causing the DNA assembly to adopt a 'closed' state at acidic pH. At neutral pH, the I-motif dissociates and entropy as well as electrostatic repulsion between the duplex arms causes the assembly to adopt an extended 'open' conformation. This forms the molecular basis of a fluorescence resonance energy transfer (FRET)-based pH sensor using the I-switch. Previous work has shown that this DNA nanomachine could function autonomously inside living cells in culture by using it to map spatiotemporal pH changes associated with endosome maturation [10] . Thus far, this represents rare evidence of quantitative functionality of a rationally designed DNA nanodevice inside cultured cells. Given the paucity of synthetic DNA nanodevices in living systems, the I-switch presents the most potential to establish the relevance of synthetic DNA nanodevices in multicellular living organisms. 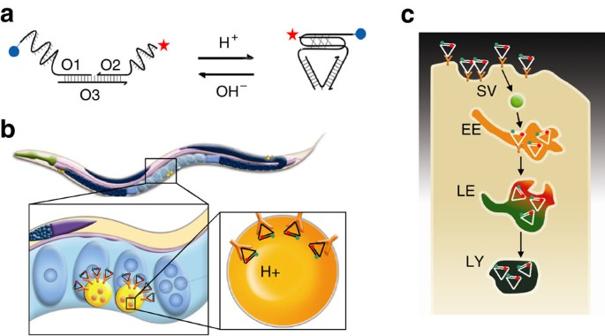Figure 1: Probing the functionality of a DNA nanomachine in coelomocytes ofC. elegans. Schematic showing (a) the structure and working of I-switch. (b) I-switch uptake in coelomocytes postinjection inC. elegans(adapted from Altun and Hall13). (c) Stages in endosomal maturation of receptor-mediated endocytosis of a ligand (SV, spherical vesicle; EE, early endosome; LE, late endosome; LY, lysosome). Figure 1: Probing the functionality of a DNA nanomachine in coelomocytes of C. elegans . Schematic showing ( a ) the structure and working of I-switch. ( b ) I-switch uptake in coelomocytes postinjection in C. elegans (adapted from Altun and Hall [13] ). ( c ) Stages in endosomal maturation of receptor-mediated endocytosis of a ligand (SV, spherical vesicle; EE, early endosome; LE, late endosome; LY, lysosome). Full size image The multicellular model organism Caenorhabditis elegans has six large scavenger cells, called coelomocytes, located in the pseudocoelomic cavity that continuously endocytose macromolecules from the body cavity. The scavenging activity of these cells has been exploited to study endocytosis in the nematode [12] . Thus, we chose this in vivo system to explore the functionality of the present DNA nanomachine ( Fig. 1b ). The present investigations revealed that DNA nanostructures are targeted to scavenger receptors (SRs) present on coelomocytes and are taken up in these cells via receptor-mediated endocytosis ( Fig. 1c ). We demonstrate herein that post endocytosis, the I-switch is functional, recapitulating its pH-sensing properties in vivo with high fidelity and shows highest dynamic range in the pH regime 5.3–6.6. This positions it to not only map spatiotemporal pH changes occurring during endosome maturation, but also other pH-dependent and pH-correlated biological events in vivo [14] . Design of the I-switch The DNA nanomachine, that is referred to as the I-switch, is composed of three DNA oligonucleotides, O1, O2 and O3, where O1 and O2 are hybridized to flanking sequences on O3, leaving a single base gap in the middle ( Fig. 1a ). The pH-responsive elements in this assembly are single-stranded cytosine-rich tracts present as overhangs on the 5′ and 3′ ends of O1 and O2, respectively [10] . At acidic pH, these cytosines form CH + · C non-Watson Crick base pairs, forming an intramolecular I-motif [11] that yields the 'closed state' of the I-switch. At neutral pH, the I-motif is dissociated and entropy as well as electrostatic repulsion drives the formation of the 'open' extended duplex conformation ( Fig. 1a ). Donor (Alexa 488) and acceptor (Alexa 647) fluorophores, that undergo FRET, are attached to O1 and O2, respectively, resulting in the assembly showing high FRET at pH 5 and low FRET at pH 7. Thus, when a solution of the doubly labelled I-switch (I A488/A647 ) is excited at the donor excitation wavelength (488 nm), the donor/acceptor (D/A) ratio shows a characteristic sigmoidal profile as a function of pH [10] . I-switch marks coelomocytes in C. elegans Coelomocytes of C. elegans are known to endocytose foreign substances injected in the body cavity [12] . To study whether the native I-switch marks coelomocytes in C. elegans , Alexa 647 labelled I-switch (I A647 ) was injected in the pseudocoelom of 1-day-old wild type hermaphrodites. After 1 h, it was seen that the I-switch specifically marks a set of six cells ( Fig. 2a ), localizing in bright punctate structures of ~0.8 μm size (Inset, Fig. 2a ). These were confirmed to be endosomes within coelomocytes ( Supplementary Fig. S1 ). 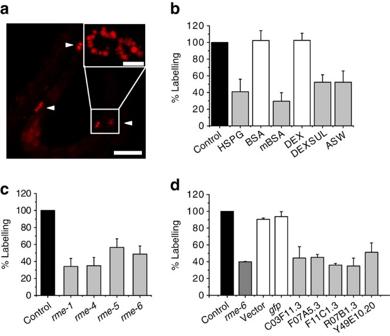Figure 2: I-switch marks endosomes of the anionic-ligand binding receptor (ALBR) pathway in coelomocytes ofCaenorhabditis elegans. (a) Epifluorescence image of wild type hermaphrodite microinjected with IA647. Arrowheads indicate labelled coelomocytes. Scale bar, 50 μm. Inset: Representative confocal image of labelled coelomocytes. Scale bar, 5 μm. Percentage of coelomocytes labelled with IA647(b) in the presence of excess competitor ligands (HSPG: heparan sulphate proteoglycan, BSA: bovine serum albumin, mBSA: maleylated BSA, DEX: dextran, DEXSUL: dextran sulphate, ASW: double-stranded DNA). Error bars represent s.e.m. (n=20 worms) (c) inrceptor-mediated endocytosis(rme)mutants. Error bars indicate s.e.m. (n=20 worms) (d) in post RNAi-mediated knockdown of the indicated gene products in hermaphrodites. Error bars represent s.e.m. (n=45 worms). Figure 2: I-switch marks endosomes of the anionic-ligand binding receptor (ALBR) pathway in coelomocytes of Caenorhabditis elegans . ( a ) Epifluorescence image of wild type hermaphrodite microinjected with I A647 . Arrowheads indicate labelled coelomocytes. Scale bar, 50 μm. Inset: Representative confocal image of labelled coelomocytes. Scale bar, 5 μm. Percentage of coelomocytes labelled with I A647 ( b ) in the presence of excess competitor ligands (HSPG: heparan sulphate proteoglycan, BSA: bovine serum albumin, mBSA: maleylated BSA, DEX: dextran, DEXSUL: dextran sulphate, ASW: double-stranded DNA). Error bars represent s.e.m. ( n =20 worms) ( c ) in rceptor-mediated endocytosis ( rme) mutants. Error bars indicate s.e.m. ( n =20 worms) ( d ) in post RNAi-mediated knockdown of the indicated gene products in hermaphrodites. Error bars represent s.e.m. ( n =45 worms). Full size image I-switch enters coelomocytes via receptor-mediated endocytosis Generally, molecules are endocytosed by cells primarily via receptor-mediated pathways or fluid-phase endocytosis [15] . It is important to determine the mode of endocytosis of the I-switch to identify the particular endocytic pathway, whose maturation-associated pH changes it would map, if any. Therefore, competition experiments were performed with ligands for receptor-mediated endocytosis (maleylated bovine serum albumin (BSA), heparan sulphate and dextran sulphate) [16] and fluid-phase markers (BSA and dextran) [12] . A solution containing I A647 and 300 equivalents of a given unlabelled competitor was injected into hermaphrodites, and the numbers of coelomocytes labelled with I A647 were counted 1 h postinjection. Interestingly, anionic molecules such as maleylated BSA (mBSA), known to bind anionic ligand-binding receptors (ALBRs) [16] , show a marked decrease in the coelomocyte labelling efficiency with I A647 . Known markers of the fluid phase, on the other hand, show no such decrease ( Fig. 2b ). Importantly, incremental increase in concentrations of mBSA shows progressively decreased labelling ( Supplementary Fig. S2a and S2b ), strongly resembling a classical binding event between a ligand and receptor [17] . Molecular genetic proof of receptor-mediated endocytosis was obtained by injecting I A647 into rceptor-mediated endocytosis ( rme ) mutants, where specific steps of receptor-mediated endocytosis pathway are compromised [18] . Compared with wild type hermaphrodites, significantly decreased labelling efficiency and labelling intensity was observed for all the rme mutants investigated ( Fig. 2c ; Supplementary Fig. S2c ). I-switch marks endosomes along the ALBR pathway It is notable that all the ligands that effectively compete with the I-switch for uptake into coelomocytes are negatively charged. Similar competition was observed between the I-switch and mBSA in Drosophila hemocytes [10] . Such negatively charged molecules function as ligands of ALBRs, also known as SRs, in both Drosophila and mammalian cells [10] , [16] . Even though worm homologues of these receptors are predicted, their function and localization is unknown. A BLASTP [19] search of the murine scavenger receptor-B (SR-B) [20] , [21] sequence against the C. elegans genome yielded six candidate genes ( Supplementary Tables S1–S3 ). Whether these SR-B candidate receptors are indeed present on coelomocytes and responsible for I-switch uptake was studied by knocking down these proteins using RNA interference (RNAi) [22] . Worms depleted of each of these candidate gene products were injected with I A647 and assayed for labelling. It was found that a reduction in the expression levels of these gene products indeed decreases labelling of coelomocytes ( Fig. 2d ; Supplementary Fig. S3b ). Consistent with the reduction in the numbers of coelomocytes labelled, a significant reduction in the labelling intensity of all vesicles was also observed ( Supplementary Fig. S3a ). This confirms that surface SR-B receptors function as ALBRs and are responsible for the uptake of I-switch ( Supplementary Fig. S4 ). Spatiotemporal mapping of pH along the ALBR pathway First, functionality of the I-switch was determined by assessing its performance quantitatively in vivo . Performance of a sensor, and consequently its integrity, is reflected by the fold change of its D/A ratio in the dynamic regime. Fold change corresponds to the value obtained by dividing the D/A ratio at the higher end of the dynamic regime to that obtained at the lower end (pH 7 and 5, respectively, in this case). To measure the fold change for the I-switch, coelomocytes were clamped at pH 5 and 7. Worms, injected with I A488/A647 , were treated with an externally added pH clamping buffer containing the ionophores nigericin and monensin to equilibrate the intra-coelomocyte pH to that of the external buffer [23] ( Supplementary Fig. S5 ). After the pH was clamped, coelomocytes were imaged and D/A ratios measured. The D/A profiles of endosomes clamped at pH 5.0 are highly characteristic and can be immediately distinguished from those clamped at pH 7.0 ( Fig. 3a ). 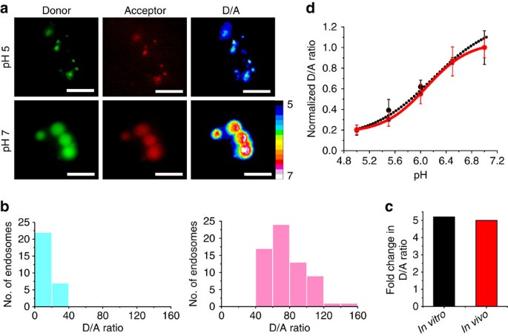Figure 3: I-switch recapitulates its pH-sensing propertiesin vivo. (a) Donor channel (D), acceptor channel (A) and respective pseudocolour D/A images of wild type coelomocytes labelled with IA488/A647and clamped at pH 5 and 7. Scale bar, 10 μm. (b) Histograms showing typical spread of D/A ratios of endosomes clamped at pH 5 (cyan) and pH 7 (pink;n=10 cells, ≥25 endosomes). (c)In vitroandin vivofold change in D/A ratios of IA488/A647at pH 7 to pH 5. (d) pH calibration curve of IA488/A647in vivo(red trace) andin vitro(black trace) showing normalized D/A ratios versus pH. Error bars indicate s.e.m. (n=25 cells, ≥50 endosomes). Figure 3b shows a histogram of a population of endosomes clamped at these pH values. This yields a fold change of ~5.0 for the I-switch in vivo . This is in excellent correspondence to the in vitro fold change, which is ~5.2 in this pH regime ( Fig. 3c ). Figure 3: I-switch recapitulates its pH-sensing properties in vivo . (a ) Donor channel (D), acceptor channel (A) and respective pseudocolour D/A images of wild type coelomocytes labelled with I A488/A647 and clamped at pH 5 and 7. Scale bar, 10 μm. ( b ) Histograms showing typical spread of D/A ratios of endosomes clamped at pH 5 (cyan) and pH 7 (pink; n =10 cells, ≥25 endosomes). ( c ) In vitro and in vivo fold change in D/A ratios of I A488/A647 at pH 7 to pH 5. ( d ) pH calibration curve of I A488/A647 in vivo (red trace) and in vitro (black trace) showing normalized D/A ratios versus pH. Error bars indicate s.e.m. ( n =25 cells, ≥50 endosomes). Full size image Given the preservation of functionality at the level of fold change, we proceeded to study the response of the I-switch over the complete pH-sensitive regime. For this, the pH was clamped at intermediate pH values (5≤pH≤7) and D/A value at each pH was plotted as a function of pH ( Fig. 3d ). The in vivo pH response curve of the I-switch shows a sigmoidal profile with highest dynamic range in the pH regime 5.3–6.6 ( Supplementary Fig. S6 ). To follow endosomal maturation of the ALBR pathway, it is necessary to first determine the temporal regimes corresponding to each stage of endosomal maturation along the pathway, that is, determine the residence times of internalized I-switch in the early endosome, the late endosome and the lysosome. Therefore, time-course experiments were performed with I A647 in hermaphrodites expressing green fluorescent protein (GFP) fused to well-known endocytic compartment markers in the coelomocytes [24] . For example, LMP-1 is a well-known marker of the lysosome [25] . Injection of I A647 in LMP-1::GFP expressing worms showed negligible colocalization 5 min postinjection ( Supplementary Fig. S7a ). The percentage colocalization steadily increased till it reached a maximum of 90% at 60 min ( Fig. 4a ; Supplementary Fig. S7b–c ). This indicates that at 1 h postinjection, endocytosed I-switch is resident mainly in the lysosomes. Similarly, using GFP::RAB-5 as an early endosomal marker [26] and GFP::RAB-7 as a late endosomal/lysosomal marker [27] , we determined that the I-switch is resident predominantly in the early and late endosomes at 5 and 17 min, respectively ( Fig. 4a ; Supplementary Fig. S7d–h ). These time points are consistent with other studies of coelomocyte endosomal maturation [24] . 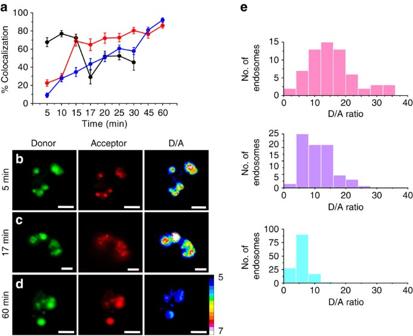Figure 4: Spatiotemporal mapping of endosomal pH changes in coelomocytes using the I-switch. (a) Trafficking of endocytosed IA647in wild type. Percentage colocalization of IA647with GFP-tagged endosomal markers (RAB-5, EE, black trace; RAB-7, LE/LY, red trace; LMP-1, LY, blue trace) at indicated times (n=10 cells, ~75 endosomes). (b, c, d) Representative pseudocolour D/A images of IA488/A647labelled coelomocytes in wild type hermaphrodites at indicated times. Scale bar, 5 μm. (e) Histograms of D/A ratios of endosomes undergoing progressive maturation, from EE at 5 min (pink) to LY at 60 min (cyan) via LE at 17 min (purple) (n=15 cells, ~100 endosomes). Figure 4: Spatiotemporal mapping of endosomal pH changes in coelomocytes using the I-switch. ( a ) Trafficking of endocytosed I A647 in wild type. Percentage colocalization of I A647 with GFP-tagged endosomal markers (RAB-5, EE, black trace; RAB-7, LE/LY, red trace; LMP-1, LY, blue trace) at indicated times ( n =10 cells, ~75 endosomes). ( b, c, d ) Representative pseudocolour D/A images of I A488/A647 labelled coelomocytes in wild type hermaphrodites at indicated times. Scale bar, 5 μm. ( e ) Histograms of D/A ratios of endosomes undergoing progressive maturation, from EE at 5 min (pink) to LY at 60 min (cyan) via LE at 17 min (purple) ( n =15 cells, ~100 endosomes). Full size image Next, I A488/A647 was injected into wild type hermaphrodites and pH measurements were made at time points of 5, 17 and 60 min ( Figs. 4b–d ), corresponding to the localization of the I-switch in the early endosome, late endosome and lysosome, respectively. Histograms of the D/A ratios of a population of endosomes at each stage are indicated in Figure 4e . It is clear that the endosomes show gradual acidification with each step. Notably, the spread in D/A ratios, and thus pH, decreases as we proceed from the early endosomes to the late endosomes and then on to the lysosomes, where the pH is relatively tightly regulated. This is consistent with other studies in the literature that have measured pH heterogeneity at different endosomal stages [28] , as well as in cellulo measurements of the same with the I-switch [10] . These D/A ratios indicate a mean pH of ~6.4 in the early endosome, ~6.0 in the late endosome and ~5.4 in the lysosome ( Table 1 ). Table 1 Mean endosomal pH at various time points post injection. Full size table Spatiotemporal pH mapping in mutants As this study shows the applicability of the I-switch in obtaining chemical information within endosomes along the ALBR-mediated endocytosis pathway, we chose two genetic backgrounds that perturb this pathway: a genetic knockout, namely rme-1 (ref. 29 ), and an RNAi knockdown, namely vha-8 (ref. 30 ). These yielded pH profiles as a function of time that were markedly different from wild type ( Table 1; Supplementary Fig. S8 ). When fluorescently labelled I-switch is injected into the pseudocoelom of C. elegans , it is seen that it is effectively uptaken exclusively by the coelomocytes. Competition experiments with different types of ligands indicate that negatively charged ligands effectively compete out I-switch uptake at the coelomocytes, implicating the presence of a receptor. This is confirmed by poor uptake in several rme mutants. RNAi knockdowns reveal that the I-switch is uptaken in coelomocytes via ALBRs. Endosomes undergo progressive acidification as they mature, from 6.0 to 6.2 in early endosomes, to ~5.5 in late endosomes and ~5.0 in lysosomes of cultured cells [28] . Given that this is well-matched with the in vitro pH sensitivity of the I-switch [10] , it could be used to map endosomal maturation along this pathway using a ratiometric approach, provided the I-switch is found to be stable as well as functional in vivo . Stability studies indicate that the I-switch has a half-life of ~8 h, which implies that even at the latest time point of measurement the I-switch is ≥95% intact ( Supplementary Fig. S9 ). The in vivo pH response profile of the I-switch exhibits remarkable correspondence with the in vitro pH calibration curve, confirming that it recapitulates its pH-sensing properties qualitatively and quantitatively in the in vivo context. Importantly, such quantitative recapitulation establishes that the sensor functions autonomously in vivo as its performance remains uncompromised, despite the molecularly complex milieu encountered therein. Given the high fidelity of the overall pH performance of the I-switch in vivo , it is possible to effectively map spatiotemporal pH changes associated with endosomal maturation of the ALBR-mediated pathway that it marks in coelomocytes. The niche of a pH-sensitive DNA nanodevice that is used as an externally introduced probe within a model organism such as C. elegans , where processes are molecularly dissected predominantly by genetics, lies in the demonstration of the nanomachine's applicability in various genetic backgrounds. rme-1(b1045) mutants have defects in recycling of receptors [29] , and show a characteristic phenotype of small indistinct cortical puncta in the coelomocytes ( Supplementary Fig. S2c ). Interestingly, the D/A distribution at the 5 and 17 min time point in rme-1 mutants show a lower spread in pH, probably due to decreased receptor recycling ( Supplementary Fig. S8c ). However, the pH of the compartments at 5 and 60 min are markedly different from wild type, suggesting alterations along the endocytic pathway at these time points ( Table 1 ). RNAi is an extremely powerful and popular tool in C. elegans to molecularly dissect pathways. Therefore, we also checked functionality of the I-switch in a vha-8 RNAi background that we predicted would perturb pH. Depletion of VHA-8 blocks V-ATPase activity, whose function is crucial for maintenance of organelle acidity [30] . Thus, perturbation of V-ATPases leads to organelles showing altered acidities [31] , [32] . Accordingly, at 5 and 17 min, the vesicles appear highly acidic ( Supplementary Fig. S8b ), showing a pH of ~5.7 and ~5.2, whereas at 60 min, the ensemble pH is ~6.0 ( Table 1; Supplementary Fig. S8d ). Thus far, under all investigated native conditions in cellulo and in vivo , the I-switch always experiences an ever-increasing acidity, where it is adopting progressively higher proportions of the 'closed' state. However, when vha-8 is depleted, the I-switch moves from a highly acidic environment to a more basic environment. This shows that the 'closed' state, once formed, can revert to the 'open' state, thus capturing the reversibility of the I-switch in a native environment in vivo . In summary, these in vivo studies unambiguously reveal that this DNA nanomachine functions autonomously in the organismal milieu. Using this DNA nanomachine, we have uncovered the existence of previously predicted cell-surface receptors and shown their involvement in uptake of DNA nanostructures in the worm. Worms injected with the I-switch remain healthy and viable ( Supplementary Fig. S10 ), showing that this DNA scaffold is non-toxic in this model system. Many pH-sensitive probes are limited by their fixed wavelengths [33] , [34] ; as the I-switch is FRET-based, it can be modulated to use FRET pairs at wavelengths that are compatible with the background of fluorescent protein-expressing transgenics. It can also be used in a range of mutant backgrounds, because it functions independently of the organismal milieu. Here, we have exploited the pH-sensitive properties of the I-switch to track pH changes associated with endosomal maturation. Many other physiological phenomena such as embryogenesis, yolk uptake, vesicular recycling, spermatogenesis, neurodegeneration, excretion and cell–cell fusion are known to be modulated by maintenance of pH homeostasis [14] and are compatible with the pH range in which the I-switch is sensitive. Because of its high sensitivity in this pH regime, the I-switch is poised to effectively capture fine changes in pH associated with these phenomena. Thus, given the utility of the I-switch, it can, in combination with other small-molecule sensors, be used to interrogate a gamut of biological processes in living organisms. In this study, for the first time, we have demonstrated quantitatively the autonomous functionality of a rationally designed, synthetic DNA nanomachine in a living organism. It is not at all obvious that functionality in a cellular milieu should imply functionality in an organismal milieu, just as in vitro functionality does not imply in cellulo functionality due to the astounding increase in molecular complexity going from the in vitro to the in cellulo context. This increase in molecular complexity is even greater on traversing the in cellulo to in vivo boundary and thus, the outcome of quantitative preservation of DNA nanodevice function in vivo is a highly encouraging finding. In addition, this particular in vivo system is a promising test bed for other DNA molecular devices [35] that can be designed to interrogate a variety of processes to track molecularly complex phenomena, thus opening up immense possibilities for the successful application of DNA nanostructures in whole organisms. Materials All fluorescently labelled high-performance liquid chromatography-purified oligonucleotides were obtained from IBA-GmBh. Unlabelled oligonucleotides were purchased from Eurofins-MWG. BSA (66 kDa), heparan sulphate (30 kDa), dextran sulphate (9,000–20,000 kDa), dextran (10,000 kDa), fluorescein isothiocyanate-dextran (70 kDa), nigericin and monensin were purchased from Sigma-Aldrich. BSA was maleylated according to a previously published protocol [36] . Trizol was purchased from Invitrogen. Sample preparation All oligonucleotides were ethanol precipitated and quantified by their ultraviolet absorbance. A sample of the I-switch was made by mixing the DNA oligonucleotides O1, O2 and O3 in equimolar ratios, heating at 90°C for 5 min, and then slowly cooling to room temperature at 5°C per 15 min. This sample preparation was carried out with oligonucleotide concentrations of 5 μM, in 10 mM phosphate buffer of pH 5.5, in the presence of 100 mM KCl. Samples were then equilibrated at 4°C overnight. Fluorescently labelled I-switch was prepared in a similar manner with fluorophore-labelled oligonucleotides. Samples were used within 7 days of annealing. C. elegans methods and strains Standard methods were followed for the maintenance of C. elegans . Wild type strain used was the C. elegans isolate from Bristol (strain N2) [37] . Mutant strains used in the study are rme-1(b1045), rme-4(b1001), rme-5(b1013) and rme-6(b1014) [18] . Transgenic strains used in this study are as follows: arIs37 [ p myo-3::ssGFP] , a transgenic strain that expresses ssGFP in the body wall muscles, which is secreted in the pseudocoelom and endocytosed by coelomocytes [12] . cdIs131 [ p cc1::GFP :: RAB-5+unc-119(+)+myo-2::GFP] , a transgenic strain expressing GFP-tagged early endosomal marker RAB-5 in the coelomocytes [24] . cdIs66 [ p cc1::GFP::RAB-7+unc-119(+)+myo-2::GFP] , a transgenic strain expressing GFP-tagged late endosomal/lysosomal marker RAB-7 in the coelomocytes [24] . pwIs50 [lmp-1::GFP+Cb-unc-119(+)] , a transgenic strain expressing GFP-tagged lysosomal marker LMP-1 (ref. 24 ). Coelomocyte labelling experiments Coelomocyte labelling, competition and rme mutant experiments were carried out with I-switch made from O2 functionalized with Alexa 647 (I A647 ). For microinjections, the I-switch sample was diluted to 100 nM in 1× Medium 1 (150 mM NaCl, 5 mM KCl, 1 mM CaCl 2 , 1 mM MgCl 2 , 20 mM HEPES, pH 7.0). Injections were performed, as previously described, in the dorsal side in the pseudocoelom, just opposite the vulva, of 1-day-old wild type hermaphrodites. Injected worms were mounted on 2.0% agarose pad and anaesthetized using 40 mM sodium azide in M9 buffer. Labelling, in all cases, was checked after 1 h of incubation at 22°C. Imaging and quantification of the number of coelomocytes labelled, in at least 20 worms, was carried out on the Zeiss Apotome. Colocalization experiments I A647 sample was diluted to 100 nM using 1X Medium 1 and injected in 10 arIs37[ p myo-3::ssGFP] hermaphrodites. Imaging and quantification of the number of coelomocytes labelled, after 1 h of incubation, was carried out on the Olympus Fluoview 1000 confocal microscope (Olympus) using an Argon ion laser for 488 nm excitation and He-Ne laser for 633 excitation with a set of dichroics, excitation, and emission filters suitable for each fluorophore. Crosstalk and bleed-through were measured and found to be negligible between GFP/Alexa 488 and Alexa 647. RNAi experiments BLASTP [19] was used to search for homologues of the murine SR-B in the C. elegans genome. Bacteria, from the Ahringer RNAi library [22] , expressing double-stranded RNA against each of the candidate genes was fed to worms, and ~45 one-day adults of the F1 progeny were assayed for labelling, by microinjections of 500 nM of I A488/A647 . The Ahringer library did not contain bacterial clones for Y76A2B.6, and hence, this gene was not assayed for I-switch uptake. mRNA levels of the candidate genes were assayed by reverse transcription–PCR. In short, total RNA was isolated using the Trizol-chloroform method; 2.5 μg of total RNA was converted to cDNA using oligo-dT primers. 5 μl of the reverse transcription reaction was used to set up a PCR using gene-specific primers. PCR products were analysed on a 1.5% agarose-TAE gel. Size of the PCR products expected for each gene were: actin (374 bp), rme-6 (847 bp), gfp (688 bp), C03F11.3 (818 bp), F07A5.3 (795 bp), F11C1.3 (898 bp), R07B1.3 (769 bp) and Y49E10.20 (777 bp). In vitro fluorescence measurements Fluorescence spectra were measured on a FluoroMax-4 instrument (Horiba Jobin Yvon). Doubly labelled I-switch (I A488/A647 ) was diluted to 100 nM in clamping buffer, the samples were excited at 488 nm and emission collected between 500–750 nm. Three independent measurements were recorded for each pH value. In vivo pH measurements pH clamping and measurement experiments were carried out with I A488/A647 . For microinjections, the I-switch sample was diluted to 500 nM using 1× Medium 1. Worms were incubated at 22°C for 1 h and then immersed in clamping buffers (120 mM KCl, 5 mM NaCl, 1 mM MgCl 2 , 1 mM CaCl 2 , 20 mM HEPES) of varying pH, containing 100 μM nigericin and 100 μM monensin [23] . To facilitate entry of the buffer into the body, the cuticle was perforated at three regions of the body using a microinjection needle [33] . After 75-min incubation in the clamping buffer, coelomocytes were imaged using wide-field microscopy. Four independent measurements, each with 10 worms, were made for each pH value. The pH clamping protocol was further verified by injecting hermaphrodites with the independent pH-sensitive probe, fluorescein isothiocyanate-dextran (70 kDa) at 1 mg ml −1 , clamping pH (with the exclusion of monensin) and imaging after 6 h. For real-time pH measurements, 10 wild type and mutant hermaphrodites were injected with I-switch and incubated at 22 °C and, after the requisite time, incubated on ice. This cold treatment efficiently stops endocytosis [24] . Worms were then anaesthetized using 40 mM sodium azide in M9 buffer and imaged on an inverted microscope. Microscopy and ratiometric image analysis Wide-field microscopy was carried out on an inverted Nikon TE2000U microscope (Nikon), equipped with mercury arc illuminator (Nikon), Photometrics Cascade II CCD camera, and dichroic and band-pass filters (Chroma Technology), suitable for the fluorophores used. Images on the same day were acquired under the same acquisition settings. All the images were background subtracted taking mean intensity over an adjacent cell-free area. Donor and acceptor images were colocalized and endosomes showing good colocalization were analysed using ImageJ ver.1.42 (NIH). Mean intensity in each endosome was measured in donor and acceptor channels. A ratio of D/A intensities was obtained from these readings. Pseudocolour images were generated by calculating the D/A ratio per pixel. Using ImageJ software, pixels were then colour coded accordingly to indicate differences between high and low D/A ratios. I-switch trafficking in coelomocytes Temporal mapping of I-switch was done in 10 worms of each of the transgenic strains mentioned above. Briefly, worms were injected with 500 nM of I A647 , incubated at 22 °C for the specified time, and then transferred onto ice. Coelomocytes were then imaged using Olympus FluoView 1,000 confocal microscope (Olympus). Colocalization of GFP and I A647 was determined by counting the numbers of I A647 -positive puncta that colocalize with GFP-positive puncta and expressing them as a percentage of the total number of I A647 -positive puncta. How to cite this article: Surana, S. et al . An autonomous DNA nanomachine maps spatiotemporal pH changes in a multicellular living organism. Nat. Commun. 2:340 doi: 10.1038/ncomms1340 (2011).